Experimental coevolution of male and female genital morphology Male genitalia typically exhibit patterns of rapid and divergent evolution, and there is now considerable evidence that sexual selection is an important driver of these patterns of phenotypic variation. Female genitalia have been less well studied, and are generally thought to be relatively invariant. Here we use experimental evolution to show that sexual selection drives the correlated evolution of female and male genital morphology in the scarabaeine dung beetle Onthophagus taurus . Moreover, we use quantitative genetic analyses to provide a rare insight into the genetic architecture underlying morphological variation in female genital morphology, and uncover evidence of the genetic covariation with male genital morphology that is expected to arise under persistent sexual selection. Male genitalia are among the most phenotypically variable of morphological traits. Sexual selection is widely believed to be responsible for this pattern of rapid and divergent evolution [1] , [2] , [3] , and there are a growing number of studies to support this view. The size or shape of a male's genitalia can influence his ability to engage the female in copula [3] , [4] , [5] , deliver his ejaculate to her reproductive tract [6] , [7] , or gain paternity of offspring she produces [8] , [9] . Male genitalia can therefore be subject to sexual selection. Macro-evolutionary studies have showed that polygamous taxa have more complex male genital morphology than monogamous taxa in which the post-copulatory processes of sexual selection, sperm competition and cryptic female choice, are unable to operate [1] . Critically, studies documenting the experimental evolution of male genital morphology have provided evidence that sexual selection underlies these macro-evolutionary patterns [3] . Cryptic female choice [2] and sexually antagonistic coevolution [10] represent two mechanisms for the evolution of genital morphology via sexual selection [11] . Cryptic female choice proposes that females bias paternity toward males whose genitalia are better able to deliver the appropriate fit and/or stimulation during copulation, and that this cryptic preference delivers indirect genetic benefits in the form of sons better equipped to gain fertilizations, and/or offspring that, on average, have a higher viability [12] . Sexually antagonistic coevolution differs from cryptic female choice in that male interests over mating, insemination and paternity are proposed to be in conflict with female interests, and impose a net fitness cost on females. Thus, male and female genitalia are argued to be subject to cycles of coevolutionary change as the sexes compete for control over mating and fertilization [10] . Critically, both mechanisms predict the coevolution of male and female genital morphology. Although there is some evidence from comparative studies of correlated patterns of evolution in male and female genital morphology [13] , [14] , [15] , [16] , [17] , [18] , and much work has explored patterns of phenotypic and genetic variation in male genital morphology [3] , [19] , few studies have focused on female genitalia. Two recent studies have suggested that female genitalia can evolve rapidly [20] and can sometimes be even more variable than male genitalia [21] . However, currently there is no direct experimental evidence that sexual selection can generate divergence in female genital morphology, or that female genitalia coevolve with male genitalia. Courting male dung beetles ( Onthophagus taurus ) mount the female and tap her dorsum and flanks with their forelimbs while reaching with their intromittent organ, the aedeagus, to make contact with her genital opening. The distal points of the aedeagus must engage with pits on the internal surface of the female's terminal segment, the pygidium, before the male can inflate his endophalus inside the female's genital tract and deliver his ejaculate [22] . Here we combine the power of experimental evolution with quantitative genetic analyses of variation in male and female genital morphology, to provide unequivocal evidence of the correlated evolution of these male and female genital structures via sexual selection. Evolutionary divergence in female genital morphology We compared morphological variation in the genital pits of females from three replicate lines of beetles that had evolved under enforced monogamy with three replicate lines that had evolved under sexual selection [23] . We sampled female beetles after 3, 13 and 19 generations of selection, and used geometric morphometric analyses [24] to capture variation in the shape and size of the genital pits, and their location on the pygidium ( Fig. 1 ). Our analysis returned 3 RW that collectively explained 75% of the shape variation; RW1 explained 43%, RW2 explained 20%, and RW3 explained 12% of the shape variation. We also extracted centroid size as an estimate of the size of the pygidium. We first determined whether centroid size had diverged in response to sexual selection, using a nested analysis of variance (ANOVA) with replicate population nested within selection history (enforced monogamy or sexual selection) as the appropriate error term. There was no significant variation due to selection history ( Supplementary Table S1 ). However, preliminary analysis suggested that the first two RW scores were significantly correlated with centroid size, indicating that shape variation may in part be explained by the size of the pygidium (Pearson's r : 0.299, P <0.001; −0.125, P =0.009; and 0.071, P =0.138, for RW 1–3 respectively; n =439). Therefore, we controlled for centroid size in all further analyses of female shape variation. We found significant divergence in RW1 ( F 1,4 =23.51, P =0.009; Supplementary Table S2 ). The genital pits decreased in circumference, moved closer together, and their distance from the outer edge of the pygidium increased in females evolving under sexual selection, whereas the reverse was true for females evolving under enforced monogamy ( Fig. 2 ). There was no significant divergence in either RW2 or RW3 ( Supplementary Table S2 ). 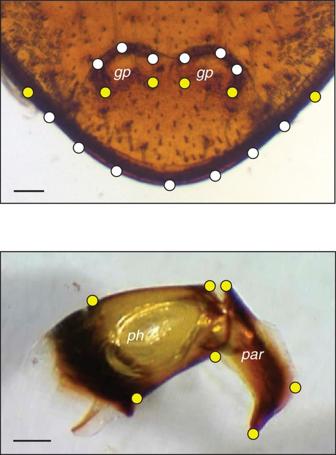Figure 1: Genital morphology ofOnthophagus taurus. Images of female (top) and male (bottom) genitalia show the placement of fixed (yellow) and semi-sliding landmarks used in the geometric morphometric analysis of size and shape variation. Note the semi-circular genital pits (gp) on the pygidium of the female, and the phalobase (ph) and parameres (par) of the aedeagus. Scale bar 0.2 mm. Figure 1: Genital morphology of Onthophagus taurus . Images of female (top) and male (bottom) genitalia show the placement of fixed (yellow) and semi-sliding landmarks used in the geometric morphometric analysis of size and shape variation. Note the semi-circular genital pits ( gp ) on the pygidium of the female, and the phalobase ( ph ) and parameres ( par ) of the aedeagus. Scale bar 0.2 mm. 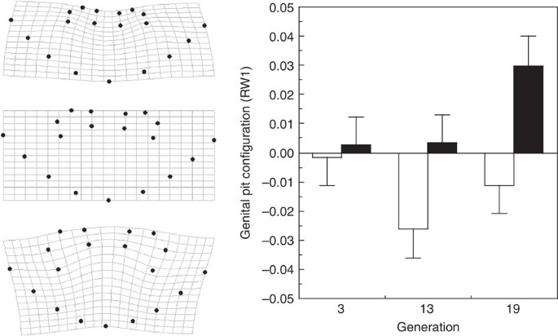Figure 2: Evolutionary divergence in female genital pit morphology. The mean (±s.e.) values of the first relative warp (RW1) are shown, pooled across 3 replicates of each treatment, measured after 3, 13 and 19 generations of experimental evolution. Lines subject to experimentally enforced monogamy are shown as open bars, and those subject or sexual selection as solid bars. Thin plate splines show the consensus shape (centre left), and extreme positive (top left) and negative (bottom left) values of the relative warp. Full size image Figure 2: Evolutionary divergence in female genital pit morphology. The mean (±s.e.) values of the first relative warp (RW1) are shown, pooled across 3 replicates of each treatment, measured after 3, 13 and 19 generations of experimental evolution. Lines subject to experimentally enforced monogamy are shown as open bars, and those subject or sexual selection as solid bars. Thin plate splines show the consensus shape (centre left), and extreme positive (top left) and negative (bottom left) values of the relative warp. Full size image Coevolutionary divergence in male genital morphology The female's genital pits and the parameres of the aedeagus are mechanically coupled during copulation [22] , and this mechanical fit might be expected to influence their mutual evolution. In a previous study, we measured the linear distances between landmarks on the aedeagus of males after 19 generations of selection, finding that the males from sexually selected lines had a longer and thinner aedeagus than males from lines evolving under enforced monogamy [3] . For our analysis of female genital morphology to be directly comparable with the data on male genital morphology, here we reanalysed the male data employing the geometric morphometric approach ( Fig. 1 ). The first three RW explained 60, 11 and 8% of the variation in aedeagus shape ( Fig. 3 ). Centroid size showed no signs of evolutionary divergence ( Supplementary Table S3 ), and significant correlations between centroid size and the RW scores suggested that aedeagus shape is in part determined by size (Pearsons r : −0.518, P <0.001; −0.158, P =0.064; and 0.299, P =0.004; for RWs 1–3 respectively; n =138). We therefore controlled for centroid size in all further analyses of aedeagus shape ( Supplementary Table S4 ). We found significant evolutionary divergence in RW3 ( F 1,4 =11.07, P =0.022) but no significant divergence in either RW1 or RW2. Males from sexually selected lines had an aedeagus that was elongated relative to males in the monogamous lines ( Fig. 3 ). 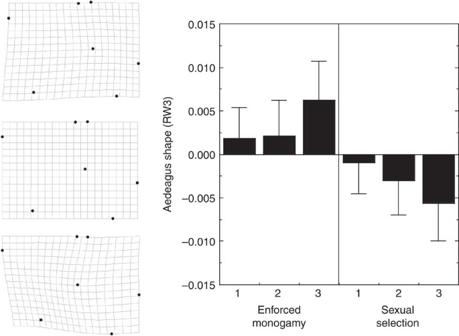Figure 3: Evolutionary divergence in male aedeagus shape. Mean (±s.e.) values of the third relative warp (RW3) after 19 generations of experimental evolution are shown for the three replicates within each enforced monogamy and sexual selection treatment. Thin plate splines show the consensus shape (centre left), and extreme positive (top left) and negative (bottom left) values of the relative warp. Figure 3: Evolutionary divergence in male aedeagus shape. Mean (±s.e.) values of the third relative warp (RW3) after 19 generations of experimental evolution are shown for the three replicates within each enforced monogamy and sexual selection treatment. Thin plate splines show the consensus shape (centre left), and extreme positive (top left) and negative (bottom left) values of the relative warp. Full size image Genetic covariance between female and male genital shape Our experimental manipulation of sexual selection in these beetles provides unequivocal evidence that sexual selection can generate an evolutionary response in the shape of both female and male genitalia. Sexual selection leads to a greater focusing and internalization of the female's genital pits, and an elongation of the male's aedeagus. The evolutionary responses we have documented here imply the existence of additive genetic variance in genital traits. More importantly, cryptic female choice and sexually antagonistic coevolution both predict the establishment of a genetic correlation between the sexes for genital shape that facilitates their correlated evolution. We used a half-sib breeding design to quantify the degree of additive genetic variation and covariation in male and female genitalia in the population used to source our experimentally evolving lines. We used the same geometric morphometric approach and, with the exception of the first relative warp for male genital morphology, found significant additive genetic variation and moderate-to-high heritabilities for male and female genital traits ( Table 1 ). There was a significant genetic correlation between the size of male and female genitalia (0.196±0.024, t 53 =8.16, P <0.001, one-sample t -test). Importantly, after controlling for genital size, the majority of genital shape variables showed significant genetic correlations across the sexes ( Table 2 ). The sign of the genetic correlation between the first relative warp of the female's genital pits and the third relative warp of the male's aedeagus was negative, indicating that selection for an increase in the internalization of the female's genital pits should drive a correlated increase in the length of the male's aedeagus ( Fig. 4 ), the exact correlated response that we observed in our experimentally evolving lines. Table 1 Quantitative genetic variance in the geometric morphometric measures of male and female genital morphology. Full size table Table 2 Matrix of genetic correlations between measures of male and female genital shape. 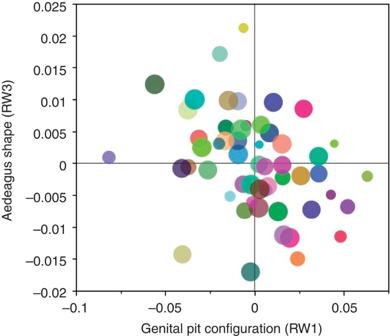Figure 4: Genetic covariance between female and male genital morphology. The bubble plot shows the sons aedeagus shape (RW3) on daughters genital pit configuration across 54 sire families. RW scores are adjusted for variation due to centroid size. Colours represent different sires, and the size of the bubbles the number of son-daughter pairs available for analysis (range 3–16). Full size table Figure 4: Genetic covariance between female and male genital morphology. The bubble plot shows the sons aedeagus shape (RW3) on daughters genital pit configuration across 54 sire families. RW scores are adjusted for variation due to centroid size. Colours represent different sires, and the size of the bubbles the number of son-daughter pairs available for analysis (range 3–16). Full size image Our data provide the first estimates of quantitative genetic variation in female genital morphology, and the first evidence of genetic covariation between male and female genitalia. Interestingly, a recent study of carabid beetles identified three quantitative trait loci for male and female genital traits that occurred almost at the same position on the genome [25] . We expect that future work will uncover close genetic associations between genes that control the development of male and female genital morphology across a broad array of animal taxa, and the correlated evolution of male and female genital traits among natural populations of the same species [26] . Some previous comparative analyses of insects and spiders have failed to find evidence for the divergent coevolution of female genital morphology [27] , [28] . However, as a recent study has shown, divergence in female genital morphology is likely to be limited to structures that physically interact with male structures [20] , as demonstrated here for the female genital pits and male parameres of onthophagine dung beetles. Moreover, female genitalia may exhibit more cryptic patterns of coevolution. If female choice of males is based on stimulation received during copulations, we would expect to see coevolution between male morphology and female sensory physiology, rather than between male and female morphology. Future studies of female genital evolution and coevolution should focus on structures that interact directly with male genitalia, and on the sensory physiology of female genital tracts [7] . Although our data provide unequivocal evidence that sexual selection drives the correlated evolution of male and female genital morphology, distinguishing between the proposed mechanisms of sexual selection is difficult [11] . Sexual conflict in our sexually selected lines may have favoured the evolution of female morphology that makes it more difficult for males to gain genital coupling, which in turn may have favoured the evolution of an elongated aedeagus that allows a male to reach the female's genital pits at a direct cost to female fitness. Alternatively, the coevolution of male and female genital morphology may be the result of females cryptically choosing males better able to engage them in copulation. The distinction lies in the costs and benefits accrued by females from mating [11] . Under sexually antagonistic coevolution, females are proposed to avoid the costs of superfluous mating by making it difficult for males to gain sexual contact. In contrast, under cryptic female choice, females are expected to gain indirect genetic benefits for offspring by mating with attractive males. In these dung beetles, the available evidence is most aligned with a mechanism of cryptic female choice, because sexual selection promotes offspring condition in our evolving lines [23] , and mating with attractive males increases the viability of offspring at no apparent cost to females [29] , [30] , [31] . Experimental evolution Full details of the source population, and the protocols adopted during experimental evolution are published elsewhere [23] . Briefly, ∼ 1,000 beetles were collected from a natural population in the south west of Western Australia and bred in the laboratory for 2 generations. Six lines were established from this laboratory stock. The effective population sizes of all lines were ∼ 100, and they differed only in the opportunity for sexual selection to operate. Under enforced monogamy, 50 females were allocated at random with 50 males to produce subsequent generations. Under sexual selection, females interacted freely with males and mated with an average of 4.5±0.2 males (range 1–8) among whom paternity was distributed equally. The opportunity for sexual selection in these lines, estimated from the standardized slope of male fitness on number of mates, the Bateman gradient, was 0.83±0.02. Lines were allowed to evolve for 19 generations. The independent units of replication in experimental evolution studies are the replicate lines ( N =3 per treatment). To obtain the appropriate error term for our analysis, we conducted nested ANOVAs with replicate population nested within treatment as a random effect. In those analyses where we sampled beetles from several generations, we included the term 'generation' and the interaction between generation and treatment. The significance of these terms was assessed relative to the random term, generation by replicate nested within treatment ( Supplementary Tables S1 and S2 ). Geometric morphometric analyses The pygidium was detached from the abdomen of the female beetle and mounted on a microscope slide with the aid of a smear of petroleum jelly. An image was captured using a Leica MZ6 binocular microscope and an AxioCam MRc5 camera (Zeiss). To capture variation in the location and shape of the genital pits on the pygidium of the female, a total of 19 landmarks, 6 fixed and 13 semi-sliding, were placed around the genital pits and the edge of the pygidium ( Fig. 1 ) using the software tpsDig2 v2.12 ( http://life.bio.sunysb.edu/morph ; F. James Rohlf, Department of Ecology and Evolution, Stony Brook University, New York). Geometric morphometric analysis determines the average positions for each landmark and calculates a consensus shape on the basis of all images of a structure. Partial warps describe variation in each landmark position of an image relative to the consensus shape, and relative warp analysis is analogous to a principal components analysis that reduces the data set to a manageable number of major axes of variation in partial warps that best describe overall shape variation. A measure of the size of the trait is obtained from the square root of the summed distances between each landmark and the average or centroid position [24] . The software Tpsrelw v1.46 was used to extract RW and centroid sizes. To assess the reliability of landmark placement, and thus the repeatability (R) of our measurements, we placed landmarks on three copies of the same image derived from each of 10 females. RW and centroid sizes were then extracted and subjected to a repeatability analysis. Our measures of genital shape and size, and thus landmark placement, were highly repeatable: the variance between subjects was greater than the variance between measures of the same subject (RW1: F 9, 20 =22.08, P <0.001, R =0.954; RW2: F 9, 20 =16.71, P <0.001, R =0.941; RW3: F 9, 20 =79.00, P <0.001, R =0.987; centroid size: F 9, 20 =163.30, P <0.001, R =0.994). For males, the aedeagus, which lies internally while not in use, was dissected from the body cavity and similarly mounted on a microscope slide for image capture. Seven fixed landmarks were placed on each image ( Fig. 1 ), and the RW and centroid sizes were extracted as described above. Landmark placement and thus measures of aedeagus size and shape were highly repeatable (RW1: F 9, 20 =22.01, P <0.001, R =0.955; RW2: F 9, 20 =16.72, P <0.001, R =0.940; RW3: F 9, 20 =78.87, P <0.001, R =0.987; centroid size: F 9, 20 =171.25, P <0.001, R =0.994). Although RW are a statistical construct, they provide a quantitative measure of biological variation in shape; unit increases in the value of a relative warp describe biological changes in shape. These can be seen from thin plate splines in Figures 2 and 3 that show the shape variation for the consensus (relative warp scores equal to zero) and extreme positive or negative values of the RW. These quantitative measures of shape can thus be used to explore quantitative differences in shape among populations, and quantitative genetic variation in genital shape. Quantitative genetic analyses We used a standard half-sib breeding design [32] to estimate patterns of additive genetic variation and covariation in male and female genitalia. For our analysis of female genitalia, we obtained 634 female offspring from 167 dams (mean±s.e., 3.8±0.11 offspring per dam, range 1–5) distributed across 55 sires (3.0±0.07 dams per sire, range 2–3). We extracted RWs and centroid sizes for each female offspring following the procedures outlined above. Shape variables were correlated with trait size (see main text), so we calculated residual RWs controlling for centroid size before calculating genetic parameters for shape. We used Restricted Maximum Likelihood procedures in S-Plus to extract quantitative genetic parameters [33] . For our analysis of male genitalia, we obtained 680 male offspring from 202 dams (3.4±0.11 offspring per dam, range 1–6) distributed across 67 sires (3.0±0.08 dams per sire, range 2–4). As for female genital shape, we controlled for centroid size in the quantitative genetic analysis of male genital shape. Finally, to estimate genetic covariances between males and females, we used the third method proposed by Via [34] . Each female offspring for which we had measures of genital shape and centroid size, was randomly assigned a full sibling male for which we also had measures of genital shape and size. We were able to generate 513 sister–brother pairs from 162 dams (3.17±0.11 pairs per dam, range 1–5) distributed across 54 sires (3.0±0.07 dams per sire, range 2–4). Variance and covariance components were estimated using Restricted Maximum Likelihood procedures implemented in S-Plus. Genetic correlations were calculated following standard procedures [35] , and their standard errors were estimated by jackknifing over sires [36] . How to cite this article: Simmons, L. W. & Garcia-Gonzalez, F. Experimental coevolution of male and female genital morphology. Nat. Commun. 2:374 doi: 10.1038/ncomms1379 (2011).